A natural mutation in the promoter ofMs-cd1causes dominant male sterility inBrassica oleracea Male sterility has been used for crop hybrid breeding for a long time. It has contributed greatly to crop yield increase. However, the genetic basis of male sterility has not been fully elucidated. Here, we report map-based cloning of the cabbage ( Brassica oleracea ) dominant male-sterile gene Ms-cd1 and reveal that it encodes a PHD-finger motif transcription factor. A natural allele Ms-cd1 PΔ−597 , resulting from a 1-bp deletion in the promoter, confers dominant genic male sterility (DGMS), whereas loss-of-function ms-cd1 mutant shows recessive male sterility. We also show that the ethylene response factor BoERF1L represses the expression of Ms-cd1 by directly binding to its promoter; however, the 1-bp deletion in Ms-cd1 PΔ−597 affects the binding. Furthermore, ectopic expression of Ms-cd1 PΔ−597 confers DGMS in both dicotyledonous and monocotyledonous plant species. We thus propose that the DGMS system could be useful for breeding hybrids of multiple crop species. Crop improvement via heterosis has long been applied to increase crop yield, adaptability, and resistance to biotic and abiotic stresses [1] , [2] . During the past few decades, heterosis utilization has revolutionized plant breeding, resulting in 3.5–200% yield increases in different crop species [3] . Male sterility is the most effective tool for heterosis utilization [3] , [4] . Genetically, there are two types of male sterility: cytoplasmic male sterility (CMS) and genic male sterility (GMS) [5] . CMS and thermosensitive/photoperiod-sensitive genic male sterility (TGMS/PGMS) have been widely applied in hybrid breeding [3] . However, these approaches suffer from several intrinsic problems. For instance, the CMS lines exhibit low hybrid seed quality and yields, low genetic diversity, and a risk of increased disease susceptibility. The TGMS/PGMS system, on the other hand, is susceptible to fluctuating climate conditions and can generate low-purity hybrid seeds [3] , [6] . Dominant genic male sterility (DGMS) is considered as a better approach for efficient utilization of heterosis [4] , considering it increases nitrogen use efficiency by allopollination (a 1:1 mixture of male-fertile and male-sterile hybrids) and is feasible for pyramiding multiple genes [4] , [7] , [8] . Therefore, identification of genes controlling DGMS phenotype and developing practical male sterility systems are important for hybrid seed production. Brassica oleracea has been cultivated for more than 3000 years. This species includes several economically important vegetable crops (known as cole vegetables), such as cabbage, cauliflower, broccoli, Brussels sprouts, kohlrabi and kale [9] . Cole vegetables have played an important role in the world food supply for centuries [10] . They were cultivated in an area of approximately 3.8 million hectares in 2021, with a total yield of 97.6 million tons, accounting for 8.32% of global vegetable production (Food and Agriculture Organization; https://www.fao.org ). In addition, B. oleracea is a precursor of B. napus and B. carinata , and thus represents an important germplasm for the improvement of oilseed crops [11] . Ogura CMS-based system has been widely applied in hybrid seed production in B. oleracea [12] . However, similar to most CMS systems, Ogura CMS lines exhibit floral bud abnormalities, reduced flower size, low hybrid seed quality and yield, low genetic diversity, and changes in important quality traits [13] , [14] . The dominant male-sterile mutant of B. oleracea 79-399-3 (whose causal locus was named Ms-cd1 ), was identified from a spring cabbage population [15] . It has normal-sized flowers and anthers but cannot produce viable pollen [15] . Using 79-399-3 as donor, DGMS lines of cabbage, broccoli, kohlrabi, and Chinese kale have been subsequently generated for their respective hybrid breeding [16] . The male sterility of these DGMS lines is quite stable in diverse genetic backgrounds; however, in very rare cases, trace amounts of pollen grains can be produced from a few anthers of Ms-cd1 heterozygous plants (HE-DGMS), enabling the production of homozygous male-sterile lines (HO-DGMS) from selfing progenies [15] . Based on this DGMS, commercial seed production systems have been developed for multiple cole vegetables [15] . Previous studies have reported molecular markers associated with Ms-cd1 and this gene was found to be located on C09 [16] , [17] . However, the gene responsible for this DGMS phenotype remains unknown. In this study, we report map-based cloning of the cabbage dominant male-sterile gene Ms-cd1 , explore the underlying molecular mechanism leading to male sterility, and propose the utilization of the system for hybrid breeding in multiple crop species. We envision that the cloned Ms-cd1 gene and its associated DGMS system can help to improve the breeding of hybrid cultivars. Dominant male-sterile phenotype of Ms-cd1 plants Plants of the Ms-cd1 dominant genic male-sterile DGMS01-20 line have normal-sized anthers but fail to produce viable pollen (Fig. 1a, b ). Similar to Arabidopsis [18] , anther development of cabbage can be divided into 14 stages (Supplementary Fig. 1a ). No obvious differences were found between wild-type (WT) 01-20 and DGMS01-20 plants before the tetrad stage (Fig. 1c and Supplementary Fig. 1a ). In the late-tetrad stage (late stage 7), DGMS01-20 plants showed delayed tapetal degeneration without a DNA fragmentation signal, as indicated by terminal transferase-mediated dUTP nick-end labeling (TUNEL) assays (Fig. 1d ). After stage 7, in 01-20, microspores were released from the tetrads through degeneration of the pollen mother cell wall and the callose wall; however, in DGMS01-20, the pollen mother cell wall failed to degenerate, and microspores became arrested in tetrads and could not be separated throughout the later developmental stages (Fig. 1c–f and Supplementary Fig. 1a ). At stage 9, DGMS01-20 microspores began to degenerate, as indicated by the DNA fragmentation signal, followed by cytoplasm vacuolation, cytoplasm degeneration and collapse (Fig. 1d and Supplementary Fig. 1a ). Severe defects in exines and intines were observed: nexines and intines were completely absent; sexines formed but were unevenly deposited, with indistinguishable tecta and bacula in some regions; and pollen coats were produced but could not be deposited on the surface of microspores (Fig. 1e, f ). Sexines were highly reduced in later stages (Fig. 1e, f ). An abnormal pollen wall structure was also observed by scanning electron microscopy (SEM) (Supplementary Fig. 1b ). At stages 13–14, DGMS01-20 anthers underwent normal dehiscence, but the microspores were morphologically degenerated (Supplementary Fig. 1a ). Fig. 1: Phenotypes and cytological characteristics of wild-type 01-20 and the DGMS01-20 mutant. a , b Comparison of flowers ( a1 , b1 ), anthers ( a3 , b3 ) and pollen grains stained with Alexander solution ( a2 , b2 ) among wild-type 01-20 and DGMS01-20 mutants. Scale bar, 3 mm in ( a1 and b1 ), 2 mm in ( a3 and b3 ), 50 μm in ( a2 and b2 ). c Transverse section analysis of anthers in the WT and DGMS01-20 mutant at S6 (stage 6), S7 (stage 7) and S9 (stage 9). E epidermis, En endothecium, ML middle layer, T tapetum, PMC pollen mother cell, Tes tetrads, Msp microspore. Scale bar, 50 μm. d TUNEL signals of anthers in the WT and DGMS01-20 mutant at stages S6, S7 and S9. White arrows indicate the TUNEL signals. Scale bar, 50 μm. e TEM analysis of microspores in the WT and DGMS01-20 mutant at anther stages S7, S9 and S10. Te tectum, Ba bacula, Nu nucleus, OCW outer cell wall. Scale bar, 4 μm. f TEM analysis of the pollen wall in the WT and DGMS01-20 mutant at anther stages S7, S9 and S11. PM microspore plasma membrane, In intine, Ne nexine. Scale bar, 2 μm. Experiments were repeated three times independently with similar results. Full size image DGMS01-20 plants were completely identical to 01-20 plants except for pollen development (Supplementary Fig. 2 ). 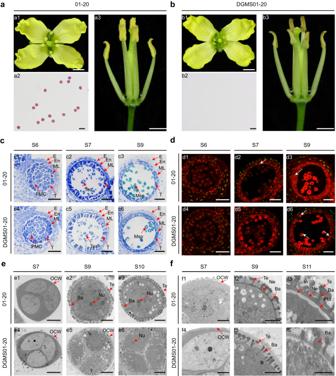Fig. 1: Phenotypes and cytological characteristics of wild-type 01-20 and the DGMS01-20 mutant. a,bComparison of flowers (a1,b1), anthers (a3,b3) and pollen grains stained with Alexander solution (a2,b2) among wild-type 01-20 and DGMS01-20 mutants. Scale bar, 3 mm in (a1andb1), 2 mm in (a3andb3), 50 μm in (a2andb2).cTransverse section analysis of anthers in the WT and DGMS01-20 mutant at S6 (stage 6), S7 (stage 7) and S9 (stage 9). E epidermis, En endothecium, ML middle layer, T tapetum, PMC pollen mother cell, Tes tetrads, Msp microspore. Scale bar, 50 μm.dTUNEL signals of anthers in the WT and DGMS01-20 mutant at stages S6, S7 and S9. White arrows indicate the TUNEL signals. Scale bar, 50 μm.eTEM analysis of microspores in the WT and DGMS01-20 mutant at anther stages S7, S9 and S10. Te tectum, Ba bacula, Nu nucleus, OCW outer cell wall. Scale bar, 4 μm.fTEM analysis of the pollen wall in the WT and DGMS01-20 mutant at anther stages S7, S9 and S11. PM microspore plasma membrane, In intine, Ne nexine. Scale bar, 2 μm. Experiments were repeated three times independently with similar results. Female fertility was normal, and the mutant could be maintained by crossing with WT plants, resulting in progeny segregating in accordance with a 1:1 (fertile:sterile) ratio (Supplementary Table 1 ). Map-based cloning of Ms-cd1 To determine the causal gene of Ms-cd1 , we employed a positional cloning approach involving three advanced backcross populations, PO1 (resulting from DGMS01-20 × 01-20; BC 24 ), PO2 (resulting from DGMS87-534 × 87-534; BC 23 ) and PO3 (resulting from DGMS18k × 18k; BC 20 ), which were developed with 79-399-3 as a donor and with backcrossing to the recurrent parents for more than 20 generations (Fig. 2a ). PO1 was used for bulked-segregant analysis sequencing (BSA-seq), and a candidate genomic region was detected within 28–31 Mb on C09 (“02-12” reference genome, version 1) (Supplementary Fig. 3 ). Polymorphic markers were developed to genotype individuals of PO1 and PO2, and Ms-cd1 was delimited to a 725-kb region. Using the segregating PO3 population (12608 individuals), we ultimately mapped Ms-cd1 to a 10.9-kb interval (Fig. 2b ). Fig. 2: Positional cloning of Ms-cd1 on chromosome 9. a Flowers from the parents of the three mapping populations. b Ms-cd1 was mapped to a ~10.9-kb interval between markers K9-31 and K9-39, and allelic variations in this genomic DNA region were evaluated. Full size image Annotations according to the “02-12” cabbage reference genome in the BRAD database ( http://brassicadb.cn ) revealed that the 10.9-kb region harbors the promoter region, the first exon and part of the first intron of Bol035718 . However, no nucleotide variation was present in the coding region of Bol035718 between the DGMS and WT plants. After sequencing the whole 10.9-kb genomic sequence, we detected only one mutation in the DGMS plants, a 1-bp deletion located 597 bp upstream of the start codon of Bol035718 (Fig. 2b ). Therefore, we speculated that this 1-bp deletion may be responsible for dominant male sterility. The expression of Bol035718 driven by the mutant promoter of DGMS plants results in dominant male sterility To verify the function of Bol035718 , a construct containing a 6,028-bp genomic fragment including the mutated promoter region (2913 bp), the Bol035718 gene (2775 bp) and the terminator region (340 bp) was generated and introduced into cabbage inbred line 01-20 by Agrobacterium -mediated transformation (Supplementary Fig. 4 ). Seven independent transgenic lines showed complete male sterility, identical to that of DGMS01-20, with normal-sized anthers, no viable pollen, microspores arrested in tetrads, an absence of pollen nexines and intines, and complete abortion of microspores that were completely aborted before stage 13 (Fig. 3a–c and Supplementary Fig. 5 ). Progeny derived from the crossing of male-sterile transgenic plants with WT 01-20 segregated in accordance with a 1:1 ratio (Fig. 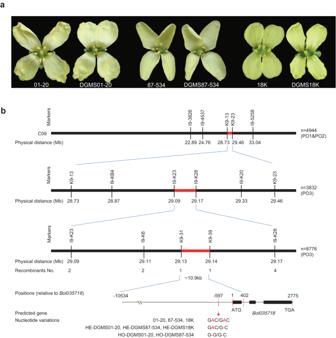Fig. 2: Positional cloning ofMs-cd1on chromosome 9. aFlowers from the parents of the three mapping populations.bMs-cd1was mapped to a ~10.9-kb interval between markers K9-31 and K9-39, and allelic variations in this genomic DNA region were evaluated. 3b and Supplementary Table 2 ). Therefore, we concluded that Bol035718 corresponds to Ms-cd1 controlling male sterility and that the 1-bp deletion upstream of Bol035718 is the causal mutation. Hereafter, the allele causing DGMS is referred to as Ms-cd1 PΔ-597 , and the WT allele is referred to as Ms-cd1 PWT . Fig. 3: Functional characterization of Ms-cd1 . a Flowers, anthers and pollen grains of WT, PΔ-597::gMs-cd1 and the ms-cd1 PWT and ms-cd1 PΔ-597 mutant plants stained with Alexander solution. Scale bar, 3 mm. b – e Transverse section, TEM, and SEM analysis of anthers in WT, PΔ-597::gMs-cd1 and the ms-cd1 PWT and ms-cd1 PΔ-597 mutant plants. E epidermis, En endothecium, ML middle layer, T tapetum, PMC pollen mother cell, Tes tetrads, Msp microspore, Te tectum, Ba bacula, In intine, Ne nexine, OCW outer cell wall. Scale bar, 50 μm in ( e1 – e3 ), ( f1 – f3 ), ( g1 – g3 ) and ( h1 – h3 ); 4 μm in ( e4 ), ( e6 ), ( f4 ), ( f6 ), ( g4 ), ( g6 ), ( h4 ) and ( h6 ); and 1 μm in ( e5 ), ( f5 ), ( g5 ) and ( h5 ). Experiments were repeated three times independently with similar results. Full size image Knocking out Ms-cd1 results in recessive male sterility different from that of the DGMS type Ms-cd1 encodes a transcription factor with a PHD-finger motif that is homologous to MS1 in Arabidopsis , PTC1/OsMS1 in rice, and ZmMs7 in maize (Supplementary Fig. 6a ) [6] , [19] , [20] , [21] , [22] . Although these homologs are reported to be involved in anther and male gamete development, mutants of the corresponding genes show recessive inheritance and cause completely different male-sterile phenotypes from those of DGMS plants observed in this study. As the only case of a natural allele with a gain of function among MS1 homologs, Ms-cd1 PΔ-597 in B. oleracea seems to play a role in a different molecular mechanism regulating male sterility. To further verify the function of Ms-cd1 , we generated a clustered, regularly interspaced, short palindromic repeats (CRISPR)/CRISPR-associated 9 (Cas9) (CRISPR/Cas9) construct in which the guide RNA targeted the third exon of Ms-cd1 (Fig. 3a ), and we transformed WT 01-20 plants with this construct. Homozygous ms-cd1 PWT mutants ( ms-cd1 PWT / ms-cd1 PWT ) were completely male sterile but with differences from the DGMS mutant, as the former produced shriveled anthers that failed to produce pollen grains at the mature stage (Fig. 3a ). The anthers and microspores of ms-cd1 PWT plants developed normally up to stage 7; after this stage, the pollen mother cell wall degenerated normally, enabling the release of microspores. These microspores formed abnormal walls and presented irregular spike-shaped bacula (rather than the rod-like bacula of the WT), thinner nexine and intine walls, and a reduced pollen coat. Moreover, microspore cytoplasm vacuolation and degeneration began soon after the release of microspores from tetrads, and complete microspore degeneration resulted in empty locules (Fig. 3d and Supplementary Figs. 5 , 7 and 8 ). Moreover, there were no differences between the ms-cd1 PWT mutants and WT 01-20 plants in terms of other agronomic traits. F 1 plants derived from ms-cd1 PWT × 01-20 were completely male fertile, and the phenotypes of the F 2 progeny resulting from selfed F 1 plants fit a 3:1 (fertile:sterile) ratio (Fig. 3d and Supplementary Table 2 ), indicating that ms-cd1 PWT is a recessive male-sterile mutant. We further knocked out Ms-cd1 in the HE-DGMS01-20 background ( Ms-cd1 PWT / Ms-cd1 PΔ-597 ). After crossing the mutated T0 plants with 01-20 followed by selfing, we obtained ms-cd1 PΔ-597 mutants ( ms-cd1 PΔ-597 / ms-cd1 PΔ-597 ). Interestingly, the ms-cd1 PΔ-597 mutant was completely identical to the ms-cd1 PWT mutant in terms of all examined phenotypic characteristics, including the inheritance of the recessive male sterility trait (Fig. 3a, e , Supplementary Figs. 5 , 7 and 8 and Supplementary Table 2 ). In summary, we concluded that (I) Ms-cd1 is required for anther and microspore development; (II) both specific promoter mutation and functional Ms-cd1 are required for Ms-cd1 PΔ-597 to trigger dominant male sterility; and (III) 79-399-3 DGMS is a gain-of-function male-sterile type whose sterility is distinguishable from that of ms-cd1 loss-of-function mutants. The expression level, but not the tissue-specific expression pattern, of Ms-cd1 is altered in DGMS plants Ms-cd1 is localized in the nucleus (Supplementary Fig. 6b ). Then, we investigated the spatial expression of the Ms-cd1 gene via qRT‒PCR and in situ hybridization (ISH) assays, which revealed that Ms-cd1 was specifically expressed in tapetal cells and microspores of anthers at stages 7–8 in both the WT and dominant genic male-sterile plants (Fig. 4a, b ). qRT‒PCR assays showed that Ms-cd1 was significantly downregulated in DGMS01-20 compared with 01-20 (Fig. 4b ). Fig. 4: Expression pattern and promoter activity of Ms-cd1 . a In situ hybridization of Ms-cd1 mRNA in anthers of WT and DGMS01-20 plants at anther stages S6–S9. Hybridization with sense probes was negative in S8. Scale bar, 100 μm. b qRT‒PCR analysis of Ms-cd1 expression in various tissues of 01-20 and DGMS01-20. c , d GUS staining of seedlings, inflorescences, siliques and anthers from representative PWT::GUS and PΔ-597::GUS Arabidopsis plants. Scale bars, 2 mm for 10-day-old seedlings, 1 cm for 28-day-old seedlings, 1 mm for inflorescences, 5 mm for siliques and 25 μm for anthers. e GUS gene expression in PWT::GUS and PΔ-597::GUS . Each dot indicates an independent transgenic line. f GUS activity in PWT::GUS and PΔ-597::GUS . Each dot indicates an independent transgenic line. g Ms-cd1 (or ms-cd1 ) expression levels in WT 01-20, DGSM01-20, ms-cd1 PWT and ms-cd1 PΔ-597 . Data are presented as the means ± SD ( n = 3 for ( b ) and ( g ), n = 10 for ( e ) and ( f )). A two-tailed unpaired t -test was used for statistical analysis. Experiments were repeated three times independently with similar results. Source data are provided as a Source Data file. Full size image We further investigated promoter activities via the analysis of transgenic Arabidopsis lines expressing the GUS reporter gene under the control of the mutated promoter ( PΔ-597 ) and WT promoter ( PWT ). GUS histochemical staining and GUS gene expression levels were determined in at least ten independent PΔ-597::GUS and PWT::GUS transgenic lines, respectively. Intriguingly, in contrast to the qRT‒PCR results, PΔ-597::GUS showed dramatically enhanced GUS activity and GUS gene expression compared with PWT::GUS , indicating that PΔ-597 shows higher promoter activity (Fig. 4b–f ). To further verify this result, ms-cd1 PΔ-597 and ms-cd1 PWT mutants were selected to investigate ms-cd1 expression. The results showed that the expression levels of ms-cd1 in ms-cd1 PΔ-597 were approximately 3-fold higher than those in ms-cd1 PWT , which further suggested that PΔ-597 presented much higher promoter activity than PWT (Fig. 4g ). Additionally, ms-cd1 (or Ms-cd1 ) expression in ms-cd1 PWT and ms-cd1 PΔ-597 was dramatically enhanced compared with that in Ms-cd1 PWT and Ms-cd1 PΔ-597 plants, suggesting that functional Ms-cd1 repressed its own expression (Fig. 4g ). Considering the observed self-repression and short-stage expression characteristics, we speculated that the transcriptional ability of Ms-cd1 could not be accurately measured by qRT‒PCR. BoERF1L regulates male fertility via the direct repression of Ms-cd1 PWT expression To investigate why the promoter mutation affected the expression of Ms-cd1 , we scanned the promoter sequence with the online tool PLACE ( http://www.dna.affrc.go.jp/PLACE/signalscan.html ), but no known cis -element was identified near the -597 bp region of the promoter. To identify the upstream regulators of Ms-cd1 , we constructed a cabbage complementary DNA (cDNA) library and applied a yeast one-hybrid (Y1H) approach to search for proteins associated with the Ms-cd1 promoter. A 66-bp WT promoter fragment (624–559 bp upstream of the Ms-cd1 start codon) was used as bait to screen the cabbage cDNA library. 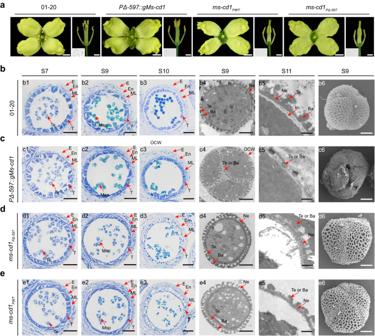Fig. 3: Functional characterization ofMs-cd1. aFlowers, anthers and pollen grains of WT,PΔ-597::gMs-cd1and thems-cd1PWTandms-cd1PΔ-597mutant plants stained with Alexander solution. Scale bar, 3 mm.b–eTransverse section, TEM, and SEM analysis of anthers in WT,PΔ-597::gMs-cd1and thems-cd1PWTandms-cd1PΔ-597mutant plants. E epidermis, En endothecium, ML middle layer, T tapetum, PMC pollen mother cell, Tes tetrads, Msp microspore, Te tectum, Ba bacula, In intine, Ne nexine, OCW outer cell wall. Scale bar, 50 μm in (e1–e3), (f1–f3), (g1–g3) and (h1–h3); 4 μm in (e4), (e6), (f4), (f6), (g4), (g6), (h4) and (h6); and 1 μm in (e5), (f5), (g5) and (h5). Experiments were repeated three times independently with similar results. Most of the positive clones (listed in Supplementary Table 3 ) obtained were derived from the same Bol028757 gene, which encodes a B. oleracea ethylene response factor 1-like (BoERF1L) transcription factor (Supplementary Fig. 9 ). To confirm the interaction between BoERF1L and the bait, we fused the full-length coding sequence of BoERF1L to the yeast GAL4 transcriptional activation domain (GAL4-AD). Ms-cd1 promoter fragments (-624 to -559) WTpro (from Ms-cd1 PWT ) and MTpro (from Ms-cd1 PΔ-597 ) (Supplementary Fig. 9 ) were inserted into the pAbAi vector as reporters. When pBoERF1L-AD was cotransformed into Y1H gold yeast cells, it significantly activated aureobasidin A (AbA) resistance in WTpro-pABAi but not MTpro-pABAi (Fig. 5a ). To confirm the binding ability, we subsequently performed an electrophoretic mobility shift assay (EMSA). The assay results showed that BoERF1L-His could directly bind WTpro but not MTpro in vitro. The unlabeled WTpro probe competed with the corresponding labeled probe and reduced the abundance of shifted bands in a concentration-dependent manner (Fig. 5b ), confirming the binding specificity of the interaction. We further divided WTpro into seven 16-bp segments, and the results showed that BoERF1L-His bound to W2-W6 but not W1 and W7 and had a higher affinity for W4 than for W2, W3, W5, and W6 (Supplementary Fig. 10 ). These data support a direct interaction between BoERF1L and the promoter of Ms-cd1 PWT from –604 to –589, with GAC as the core binding sequence, however, in the Ms-cd1 PΔ-597 promoter, the 1-bp deletion prevented this binding ability. Finally, a quantitative dual-luciferase transactivation assay (dual-LUC) was conducted to confirm the effects of BoERF1L on Ms-cd1 PWT transcription. A constitutively expressed Renilla luciferase gene driven by the 35S promoter was used as an internal reference reporter. The dual-LUC assay results showed that the BoERF1L effector strongly repressed PWT::LUC reporter transcription, whereas the negative control did not (Fig. 5c ). Taken together, these results indicated that BoERF1L directly binds to the specific site of the Ms-cd1 PWT promoter and represses Ms-cd1 PWT expression. Fig. 5: BoERF1L regulates male fertility by the direct repression of Ms-cd1 expression. a Yeast one-hybrid assay. WTpro represents a 66-bp probe (–624 to –559 upstream of ATG) from the WT promoter. MTpro represents a 65-bp probe (–624 to –559 upstream of ATG) from the DGMS01-20 promoter. Yeast strains were cultured on SD/-Leu medium with 200 ng/mL AbA. b EMSA analysis. The biotin-labeled probes are indicated. Competition for BoERF1L binding was performed with excess unlabeled WTpro probe at 20×, 30× and 40× the amount of labeled probe. c The dual-luciferase transient expression assay shows that BoERF1L represses transcription of the Ms-cd1 PWT gene promoter. Luciferase intensity was imaged and quantified using a Tanon 5200 system. d qRT‒PCR analysis of BoERF1L expression in various tissues of 01-20. e Flowers, anthers and pollen grains stained with Alexander solution among WT and boerf1l mutants. Scale bars, 3 mm for flowers, 2 mm for anthers, 50 μm for pollen grains. f , g Transverse section, TEM and SEM analysis of anthers in WT and the boerf1l mutant. E epidermis, En endothecium, ML middle layer, T tapetum, Tes tetrads, Msp microspore, Te tectum, Ba bacula, In intine, Ne nexine. Scale bars, 50 μm in ( f1 – f6 ); 4 μm in ( g1 ), ( g2 ), ( g4 ) and ( g6 ); 2 μm in ( g2 ) and ( g5 ). Data are presented as the means ± SD ( n = 10 for ( c ), n = 3 for ( d )). A two-tailed unpaired t -test was used for statistical analysis. Experiments were repeated three times independently with similar results. Source data are provided as a Source Data file. Full size image BoERF1L is highly expressed in anthers before stage 9 (Fig. 5d ). To determine whether BoERF1L plays a role in anther and microspore development, we knocked out BoERF1L by the CRISPR/Cas9 method in the 01-20 background (Supplementary Fig. 11a, b ). The boerf1 mutants showed significantly reduced male fertility, with approximately 50% pollen viability (Fig. 5e, f and Supplementary Fig. 11c ). Transmission electron microscopy (TEM) and SEM assays showed that, as in the DGMS lines, many microspores could not produce intine walls (Fig. 5g ). We further knocked down BoERF1L via RNA interference (RNAi) in the 01-20 background. Two representative lines (RNAi-4 and RNAi-6) were selected from eight independent lines for detailed studies (Supplementary Fig. 12a–c ). These lines showed a similar phenotype to the boerf1 mutants, with pollen viability of 61.2% for RNAi-4 and 56.6% for RNAi-6 (Supplementary Fig. 12d, e ). In addition, we assessed the expression of Ms-cd1 and its closely related genes in boerf1 , which showed that all the evaluated genes presented expression level alterations identical to those in the DGMS lines (Supplementary Figs. 11d and 13 ). These results suggested that BoERF1L affected the male fertility of B. oleracea via the regulation of Ms-cd1 . Ms-cd1 PΔ-597 and Ms-cd1 loss-of-function alters the expression of genes required for tapetum and pollen development As MS1 (the ortholog of Ms-cd1 ) is reported to be involved in the DYT1 - TDF1 - AMS - MS188 - MS1 network, which is critical for anther and pollen development [23] , [24] , we investigated the expression of these genes and their downstream targets. Most of them showed contrary expression levels in DGMS01-20 and ms-cd1 (Supplementary Fig. 13 ). The upstream genes BoTDF1 , BoAMS and BoMS188 were downregulated in DGMS01-20, but upregulated in ms-cd1 , indicating that Ms-cd1 played a feedback repression role in the BoDYT1 - BoTDF1 - BoAMS - BoMS188 - Ms-cd1 module. The BoQRTs genes, required for tetrad wall degeneration, and the BoTEK gene, required for pollen wall assembly were dramatically downregulated in DGMS01-20, consistent with the defects of microspore arrest in tetrads, identical to what occurs in the qrt mutant [25] , and absent nexine and intine layers, similar to what occurs in the tek mutant [26] (Fig. 1 and Supplementary Fig. 13a ). Other pollen wall development requiring genes, such as BoYP704B1 , BoPKSA , and BoPKSB were also downregulated in DGMS01-20 and upregulated in ms-cd1 . Interestingly, pollen coat-related genes such as BoLTPs , BoEXLs and BoGRPs were upregulated in DGMS01-20 and downregulated in ms-cd1 , indicating that Ms-cd1 may be an activator of pollen coat development (Supplementary Fig. 13a ). Based on the above results, a working model of the regulation of male fertility by Ms-cd1 is proposed (Supplementary Fig. 13b ). Ms-cd1 is directly targeted by the transcription factor BoERF1L to precisely maintain a stable expression level, which is essential for the feedback regulation of the BoDYT1 - BoTDF1 - BoAMS - BoMS188 - Ms-cd1 network and a subsequent series of genes required for pollen development. In DGMS, promoter mutation causes dysregulation of Ms-cd1 and strong negative feedback of the BoDYT1 - BoTDF - BoAMS - BoMS188 - Ms-cd1 module and, subsequently, pollen wall development-related genes such as BoQRTs , BoTEK and BoPKSA . In RGMS, ms-cd1 cannot feed back into the module, which results in the upregulation of some genes, such as BoTEK and BoPKSA , and the downregulation of other genes related to pollen development, such as BoLTPs and BoEXLs . Overall, our results suggest that the precise regulation of Ms-cd1 is vital for male fertility. A DGMS system for heterosis utilization in dicotyledonous and monocotyledonous crop species To further test whether Ms-cd1 PΔ-597 can induce male sterility in other plant species, we introduced PΔ-597::Ms-cd1 into Arabidopsis ecotype Columbia (Col-0), rapeseed (Westar), tomato (Ailsa Craig, AC) and rice (ZH11). More than five transgenic lines were generated for each plant species; these PΔ-597::Ms-cd1 lines exhibited normal vegetative morphology and female fertility identical to those of their corresponding WT plants but showed stable male sterility, produced no viable pollen and failed to produce seeds upon selfing (Fig. 6a–d ). 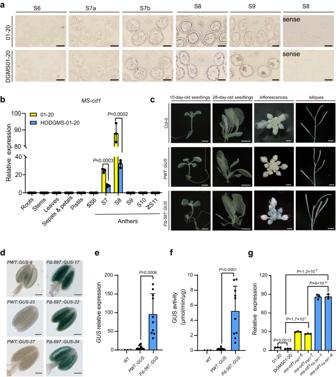Fig. 4: Expression pattern and promoter activity ofMs-cd1. aIn situ hybridization ofMs-cd1mRNA in anthers of WT and DGMS01-20 plants at anther stages S6–S9. Hybridization with sense probes was negative in S8. Scale bar, 100 μm.bqRT‒PCR analysis ofMs-cd1expression in various tissues of 01-20 and DGMS01-20.c,dGUSstaining of seedlings, inflorescences, siliques and anthers from representativePWT::GUSandPΔ-597::GUS Arabidopsisplants. Scale bars, 2 mm for 10-day-old seedlings, 1 cm for 28-day-old seedlings, 1 mm for inflorescences, 5 mm for siliques and 25 μm for anthers.eGUSgene expression inPWT::GUSandPΔ-597::GUS. Each dot indicates an independent transgenic line.fGUSactivity inPWT::GUSandPΔ-597::GUS. Each dot indicates an independent transgenic line.gMs-cd1(orms-cd1) expression levels in WT 01-20, DGSM01-20,ms-cd1PWTandms-cd1PΔ-597. Data are presented as the means ± SD (n= 3 for (b) and (g),n= 10 for (e) and (f)). A two-tailed unpairedt-test was used for statistical analysis. Experiments were repeated three times independently with similar results. Source data are provided as a Source Data file. Progenies derived from a cross between PΔ-597::Ms-cd1 and WT plants segregated at a 1:1 (fertile:sterile) ratio (Supplementary Table 4 ). The results indicated that ectopic expression of Ms-cd1 PΔ-597 induced dominant male sterility and was conserved in dicotyledonous and monocotyledonous plants. Fig. 6: Ms-cd1 PΔ-597 -induced dominant male sterility is conserved in dicotyledonous and monocotyledonous plants. a – d Flowers/anthers (scale bars, 1 mm in ( a ), 4 mm in ( b ), 2 mm in ( c and d )), pollen grains stained with Alexander solution or I2-KI solution (scale bars, 50 μm), and seed setting upon selfing among wild-type and PΔ-597::Ms-cd1 transgenic lines of Arabidopsis Col-0, rice ZH11, rapeseed Westar and tomato Ailsa Craig (AC) (scale bars, 1 cm). e Workflow of the DGMS system for heterosis utilization in cabbage. Haploid/DH inducers play a key role in the creation and propagation of HO-DGMS lines. Experiments were repeated three times independently with similar results. Full size image Exploiting male sterility to increase crop yields is feasible and vital globally. In contrast to other male sterility systems, the DGMS system has greater value, with the advantages of increasing crop yields, good efficiency and safety to the ecosystem [4] . The currently applied Ms-cd1 PΔ-597 DGMS system poses disadvantages including difficulties in generating, propagating and preserving HO-DGMS lines. Herein, we propose the following five steps for using the DGMS system. The detailed strategy is shown in Fig. 6e , with cabbage as an example. Step 1: generation of HE-DGMS lines. The DGMS gene is introduced from a donor plant to an elite line by backcrossing for 4–5 generations, or a DGMS mutant is directly generated via precise genome editing of the Ms-cd1 PΔ-597 promoter and elimination of transgene elements in Step 2. Step 2: generation and propagation of HO-DGMS lines by in vivo doubled haploid (DH)/haploid induction. First, HE-DGMS lines are pollinated with pollen from a DH/haploid inducer, such as the DH inducer Y3380 [27] and dmp -based haploid inducer [10] . Among the progeny, DHs/haploids can be identified by phenotypic markers, molecular markers or fluorescent markers. When using haploid inducers, haploids must be converted to DH plants via colchicine (or other methods). For the propagation of HO-DGMS lines, the cross-pollination of HO-DGMS and DH/haploid inducer lines can be performed by using pollinators in protected fields. Step 3: large-scale reproduction of a 100% HE-DGMS line. By crossing HO-DGMS with its corresponding maintainer line, breeders can obtain HE-DGMS lines with 100% male-sterile plants. This DGMS system requires only a few HO-DGMS plants, which can be easily produced by DH/haploid inducer lines with typical haploid induction rates of 1%~10% (taking cabbage as an example, by crossing with the maintainer line and then crossing with the male parent, one HO-DGMS plant would produce 5000 HE-DGMS individuals, and approximately 25 million F 1 seeds, which is sufficient to cultivate an area of 400 ha). Step 4: hybrid seed production. Hybrid seeds can be obtained by crossing the HE-DGMS line with another elite male parent. Step 5: crop production. For crops whose vegetative organs are harvested (e.g., cabbage), F 1 hybrids are cultivated and harvested in the same manner as traditional hybrids (Fig. 6e ). For crops whose fruits (e.g., tomato) or seeds are harvested (e.g., maize, rice), F 1 hybrids consist of 50% male-fertile plants and 50% male-sterile plants; when both types are planted in the field, the pistils of male-sterile plants can be pollinated by male-fertile plants; this allopollination promotes increased energy allocation to female organs and thereby increases crop yields [4] . Using cabbage lines HE-DGMS01-20 and HE-DGMS21-3, we generated and propagated HO-DGMS lines using dmp -based inducer lines (Fig. 7a–d ). When the lines were used for hybrid seed production, we observed that hybrid seed yields increased by more than 98% compared with those of hybrids developed via the traditional CMS-based method, and F 1 cabbage hybrids showed high quality and uniformity (Fig. 7e, f and Supplementary Fig. 14a, b ). Fig. 7: The cabbage hybrid Zhonggan 21 produced via the DGMS-based system and the DGMS-based system enhances hybrid seed yield compared with the commonly used CMS-based system. a Detection of haploid HO-DGMS from progenies of the HE-DGMS01-20 × boc03.dmp9 inducer line using KASP marker K9-6. boc03.dmp9 inducer line, a maternal haploid inducer line created previously [15] . K9-6, a KASP marker developed based on the causal mutation (–597 upstream of the start codon) of Ms-cd1 PΔ-597 . Green dots, homozygous DGMS individuals (i.e., haploid HO-DGMS01-20); red dots, heterozygous DGMS individuals; blue dots, homozygous wild-type individuals; gray dot, negative control. b Detection of haploid HO-DGMS from progenies of the HO-DGMS01-20 × boc03.dmp9 inducer line using the KASP marker K9-6. c Phenotypes of haploid and diploid HO-DGMS01-20. Diploid HO-DGMS01-20 plants were produced from haploid HO-DGMS01-20 via colchicine. Scale bars, 5 cm. d Female parent DGMS01-20, male parent 87-534 and hybrid Zhonggan 21. DGMS01-20 is generated by a dmp -based inducer. e Comparison of inflorescences and seed setting performance of the 01-20, DGMS01-20 and CMS01-20 lines. f Silique number, seed number and seed yield of DGMS01-20 and CMS01-20 lines, when crossed to the male parent 87-534. Three field replicates were performed. For each field experiment, 330 female DGMS01-20 and 165 male 87-534 were planted in a 100-m 2 area. Female plants were pollinated by honey bees ( Apis mellifera ligustica ). Thirty female individuals were randomly selected for the calculation of silique numbers and seed numbers. Seeds were harvested and weighed from all female individuals in each field experiment. Data are presented as the means ± SD ( n = 3 for ( f )). A two-tailed unpaired t -test was used for statistical analysis. 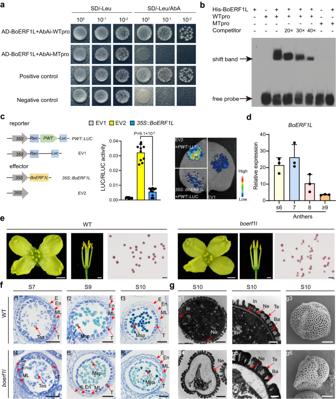Fig. 5: BoERF1L regulates male fertility by the direct repression ofMs-cd1expression. aYeast one-hybrid assay. WTpro represents a 66-bp probe (–624 to –559 upstream of ATG) from the WT promoter. MTpro represents a 65-bp probe (–624 to –559 upstream of ATG) from the DGMS01-20 promoter. Yeast strains were cultured on SD/-Leu medium with 200 ng/mL AbA.bEMSA analysis. The biotin-labeled probes are indicated. Competition for BoERF1L binding was performed with excess unlabeled WTpro probe at 20×, 30× and 40× the amount of labeled probe.cThe dual-luciferase transient expression assay shows that BoERF1L represses transcription of theMs-cd1PWTgene promoter. Luciferase intensity was imaged and quantified using a Tanon 5200 system.dqRT‒PCR analysis ofBoERF1Lexpression in various tissues of 01-20.eFlowers, anthers and pollen grains stained with Alexander solution among WT andboerf1lmutants. Scale bars, 3 mm for flowers, 2 mm for anthers, 50 μm for pollen grains.f,gTransverse section, TEM and SEM analysis of anthers in WT and theboerf1lmutant. E epidermis, En endothecium, ML middle layer, T tapetum, Tes tetrads, Msp microspore, Te tectum, Ba bacula, In intine, Ne nexine. Scale bars, 50 μm in (f1–f6); 4 μm in (g1), (g2), (g4) and (g6); 2 μm in (g2) and (g5). Data are presented as the means ± SD (n= 10 for (c),n= 3 for (d)). A two-tailed unpairedt-test was used for statistical analysis. Experiments were repeated three times independently with similar results. Source data are provided as a Source Data file. Experiments were repeated three times independently with similar results. Source data are provided as a Source Data file. Full size image Together, the stable Ms-cd1 PΔ-597 gene and its associated DGMS system are applicable for hybrid seed production in crops. As an effective pollen control tool for cross-pollination and heterosis utilization, male sterility is considered one of the most important traits extensively studied in plants [28] , [29] . However, only a few genes controlling male sterility have been identified in B . oleracea [30] . In particular, the Ms-cd1 DGMS B. oleracea line (79-399-3 mutant) is a valuable male-sterile genetic resource that has been applied to cole vegetable breeding and seed production in China. However, the Ms-cd1 gene has not been identified [16] . In this study, using a positional cloning approach, we cloned Ms-cd1 . We show that Ms-cd1 encodes a PHD-finger transcription factor, and its orthologs have been identified in several plant species: MS1 in Arabidopsis [19] , [20] , OsMs1/OsPTC1 in rice [21] , [31] , and ZmMs7 in maize [6] , [22] . Loss of function of Ms-cd1 orthologs results in recessive male sterility, similar to that of the ms-cd1 mutant in this study, indicating that Ms-cd1 plays a conserved role in regulating male reproductive development in both dicots and monocots. Among its orthologs, Ms-cd1 PΔ-597 is a unique natural dominant male-sterile allele resulting from a mutation in the noncoding region and conferring a unique mutant phenotype to anthers and microspores. The special promoter mutation and functional coding region of Ms-cd1 PΔ-597 are necessary for the Ms-cd1 gene to cause male sterility, as the ms-cd1 PΔ-597 loss-of-function allele is identical to ms-cd1 PWT . Arabidopsis MS1 functions downstream of MS188 and is involved in the well-known DYT1-TDF1-AMS-MS188-MS1 network, a feed-forward module regulating tapetum and pollen wall development by targeting a series of genes, such as QRTs , EXLs , CYP703A2 , TEK , and MS2 [23] , [24] , [26] , [32] . Nevertheless, the precise molecular mechanism of MS1 in this module remains largely unknown. Ms-cd1 PΔ-597 alters the expression of genes required for tapetum and pollen development, including its upstream genes in the DYT1-TDF1-AMS-MS188-MS1 module, indicating that Ms-cd1 is involved in negative feedback regulation of this network. Consistent with the downregulation of BoQRTs and BoTEK , DGMS plants showed some key defects similar to what is observed in the qrt mutant (microspores arrested in tetrads) [25] , [33] and the tek mutant (absence of nexine and intine layers of microspores) [26] . It will be interesting to investigate how Ms-cd1 is involved in the feedback regulation of DYT-TDF-AMS-MS188- Ms-cd1 in the future. Ethylene response factors (ERFs) belong to the plant-specific APETALA 2 (AP2) superfamily [34] . As transcription factors that respond to ethylene signals, ERFs play important roles in plant development and the response to both pathogen attack and abiotic stresses through specific binding to GCC-boxes (AGCCGCC) and DRE/CRT core motifs (A/GCCGAC) in the promoter of downstream genes [35] , [36] . Interestingly, we identified the ERF transcription factor BoERF1L, which directly binds to a motif with a GAC-core sequence in the promoter of Ms-cd1 PWT , as confirmed by the results of our in vivo and in vitro assays. Arabidopsis ERF1, an ortholog of BoERF1L, serves as a key integrator of the ethylene and jasmonic acid pathways involved in regulating the defense response and plant development [37] , [38] . In B. oleracea , BoERF1L represses the expression of Ms-cd1 PWT through its ability to bind to the GAC-core motif in the Ms-cd1 PWT promoter. This binding ability is disrupted by the 1-bp deletion in the promoter of Ms-cd1 PΔ-597 , causing dysregulation of Ms-cd1 and, ultimately, male sterility. In addition, knocking down the BoERF1L gene resulted in reduced male fertility, further confirming its role in male gamete development. These results suggest a molecular mechanism through which BoERF1L plays an important role in the precise regulation of Ms-cd1 and the maintenance of male fertility. DGMS is an ideal tool for plant breeding and seed production, with advantages including increases in production through all methods of pollination, cost effectiveness without the need for seed sorting, and feasibility of its use in hybrid breeding to pyramid multiple genes [4] , [7] . To facilitate the use of the DGMS gene Ms-cd1 PΔ-597 in crop plants, we introduced it into other plant species, which resulted in stable dominant male sterility in rice, Arabidopsis , tomato, and rapeseed, indicating that Ms-cd1 PΔ-597 - induced dominant male sterility is conserved in both dicotyledonous and monocotyledonous plants. Considering that Ms-cd1 is evolutionarily conserved in plant species [21] , [22] , DGMS plants can be directly generated by promoter modification in various crop species (especially for those without DGMS mutants) via genome editing technology. Therefore, Ms-cd1 PΔ-597 and its orthologs have great potential for hybrid breeding and seed production in multiple crop species. However, the lack of efficient systems has limited the utilization of DGMS lines. Currently, two types of DGMS systems have been developed: biotechnology-based male sterility systems (which have been used in several cereal crop species) and the Ms-cd1 PΔ-597 DGMS system (which has been used in cole vegetables) [6] , [8] , [15] . Biotechnology-based male sterility systems produce DGMS female lines and hybrids containing transgenic elements, which are regulated and limited in some countries [4] . However, the Ms-cd1 PΔ-597 DGMS system presents two disadvantages: (1) it is difficult to generate HO-DGMS plants, because it relies on the occurrence of trace amounts of pollen grains from HE-DGMS plants, and (2) HO-DGMS plants must be preserved and propagated by tissue culture, which is inconvenient and expensive [16] . By exploiting the in vivo DH/haploid induction methods, we proposed an advanced DGMS system in which an HO-DGMS line can be generated, propagated and preserved by seed. Overall, this system is transgene element free, simple, cost effective, and applicable to multiple crop species. The results of a field test showed that, compared with the CMS system, the DGMS system increased hybrid cabbage seed yield by 98%. We believe that the application of this system can also increase the yield of grain and other crop species whose seeds are harvested as products. In addition, DGMS lines can be used to integrate and pyramid multiple elite traits, such as high yield and resistance to abiotic and biotic stresses, in recurrent selection breeding. In conclusion, we report the cloning of Ms-cd1 and elucidate that it is regulated by BoERF1L to control male fertility in a dominant manner in cabbage. Based on this, we propose a DGMS system for hybrid seed production. The Ms-cd1 gene and its associated DGMS system may facilitate hybrid breeding in B. oleracea and other major crop species. Plant materials and growing conditions We used 10 cabbage ( B. oleracea var. capitata ) lines, 3 cabbage advanced backcross populations, 2 cabbage hybrids, 1 Arabidopsis thaliana line, 1 rice ( Oryza sativa L. ssp. japonica “ZH11”) line, 1 tomato ( Solanum lycopersicum “Ailsa Craig”) line, 1 rapeseed ( B. napus “Westar”) line, and 1 Nicotiana benthamiana line in this study. These plant materials and transgenic lines and the gene editing lines generated from them are listed in Supplementary Data 1 . These plant materials were grown at the Institute of Vegetables and Flowers, Chinese Academy of Agricultural Sciences, in Beijing. All cabbage plants were grown in open fields from August to mid-October and then transplanted to greenhouses. After vernalization under cold conditions (0–10 °C), they flowered in April of the following year. All rice, tomato, and rapeseed plants were grown and maintained regularly in the experimental field under local growing conditions in Beijing, China. A. thaliana Col-0 and N. benthamiana were planted in the soil and maintained in growth chambers under long-day conditions (16 h light, 8 h dark) at 22 °C. Transgenic Arabidopsis plants were screened via 1/2-strength Murashige and Skoog media supplemented with 30 mg/L hygromycin B. The hygromycin-resistant seedlings were transplanted to soil and grown under the same conditions as the WT plants. Phenotypic characterization of plant materials Images of whole plant, flower, silique, inflorescence and fruit morphology were captured with a Canon EOS M6 digital camera (Canon, Tokyo, Japan). 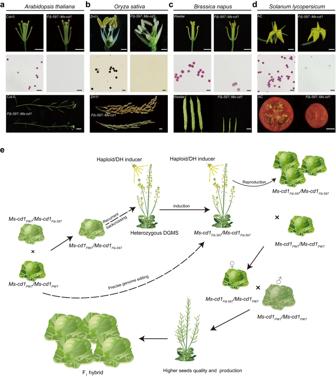Fig. 6:Ms-cd1PΔ-597-induced dominant male sterility is conserved in dicotyledonous and monocotyledonous plants. a–dFlowers/anthers (scale bars, 1 mm in (a), 4 mm in (b), 2 mm in (candd)), pollen grains stained with Alexander solution or I2-KI solution (scale bars, 50 μm), and seed setting upon selfing among wild-type andPΔ-597::Ms-cd1transgenic lines ofArabidopsisCol-0, rice ZH11, rapeseed Westar and tomato Ailsa Craig (AC) (scale bars, 1 cm).eWorkflow of the DGMS system for heterosis utilization in cabbage. Haploid/DH inducers play a key role in the creation and propagation of HO-DGMS lines. Experiments were repeated three times independently with similar results. 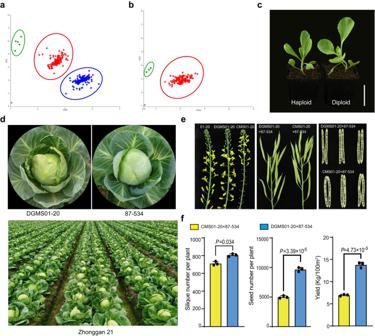Fig. 7: The cabbage hybrid Zhonggan 21 produced via the DGMS-based system and the DGMS-based system enhances hybrid seed yield compared with the commonly used CMS-based system. aDetection of haploid HO-DGMS from progenies of the HE-DGMS01-20 ×boc03.dmp9inducer line using KASP marker K9-6.boc03.dmp9inducer line, a maternal haploid inducer line created previously15. K9-6, a KASP marker developed based on the causal mutation (–597 upstream of the start codon) ofMs-cd1PΔ-597. Green dots, homozygous DGMS individuals (i.e., haploid HO-DGMS01-20); red dots, heterozygous DGMS individuals; blue dots, homozygous wild-type individuals; gray dot, negative control.bDetection of haploid HO-DGMS from progenies of the HO-DGMS01-20 ×boc03.dmp9inducer line using the KASP marker K9-6.cPhenotypes of haploid and diploid HO-DGMS01-20. Diploid HO-DGMS01-20 plants were produced from haploid HO-DGMS01-20 via colchicine. Scale bars, 5 cm.dFemale parent DGMS01-20, male parent 87-534 and hybrid Zhonggan 21. DGMS01-20 is generated by admp-based inducer.eComparison of inflorescences and seed setting performance of the 01-20, DGMS01-20 and CMS01-20 lines.fSilique number, seed number and seed yield of DGMS01-20 and CMS01-20 lines, when crossed to the male parent 87-534. Three field replicates were performed. For each field experiment, 330 female DGMS01-20 and 165 male 87-534 were planted in a 100-m2area. Female plants were pollinated by honey bees (Apis mellifera ligustica). Thirty female individuals were randomly selected for the calculation of silique numbers and seed numbers. Seeds were harvested and weighed from all female individuals in each field experiment. Data are presented as the means ± SD (n= 3 for (f)). A two-tailed unpairedt-test was used for statistical analysis. Experiments were repeated three times independently with similar results. Source data are provided as a Source Data file. Rice and Arabidopsis anthers were imaged with a SZX2-ILLB16 stereomicroscope (Olympus, Tokyo, Japan). To evaluate pollen viability, anthers of three representative individuals were analyzed. Pollen grains from dicotyledonous species, including cabbage, tomato, rapeseed, and A. thaliana , were stained with Alexander’s solution, and grains from rice plants were stained with 1% I2-KI solution and imaged with a BX-53TR microscope (Olympus, Tokyo, Japan). Darkly stained, round pollen grains were defined as viable, whereas unstained, lightly stained and irregular pollen grains were defined as sterile. For transverse section analysis, fresh anthers of B. oleracea at different developmental stages were sampled, fixed in formalin‒acetic acid‒alcohol (FAA) solution (a mixture of 37% formaldehyde, 70% ethanol, and 100% acetic acid), dehydrated through an ethanol series (70%, 85%, 95%, and 100%), subjected to transverse sectioning, embedded and cut into 2-μm sections using a Leica RM2265 microtome (Leica, Germany). The sections were further stained with 0.05% toluidine blue O and observed under a BX-51TRF microscope (Olympus, Tokyo, Japan). For SEM analysis, the anthers were fixed and dehydrated through an ethanol series (50%, 70%, 80%, 90%, and 100%), using the critical-point drying method, and then coated with gold and imaged using a scanning electron microscope (HITACHI HT7700, Japan). For TEM analysis, anthers were washed in 0.1 M phosphate buffer and embedded in epoxy resin. Ultrathin sections (50–70 nm) were cut using a Leica EM UC7 ultramicrotome (Leica Microsystems, Belgium) and stained with uranyl acetate and lead citrate. Sections were imaged using a transmission electron microscope (HITACHI, Regulus 8100, Japan). For TUNEL assays, anthers at different developmental stages were collected from WT 01-20 and DGMS01-20 plants. DNA fragmentation was detected via TUNEL assays using a TUNEL kit (G1502, Servicebio) according to the manufacturer’s instructions. The samples were subsequently evaluated under a fluorescence microscope (Nikon Eclipse C1; Nikon, Tokyo, Japan). Map-based cloning of Ms-cd1 The male-sterile lines HE-DGMS01-20, HE-DGMS87-534, and HE-DGMS18K were used as female parents in crosses with their corresponding maintainer lines to generate three advanced backcross populations: PO1 (resulting from HE-DGMS01-20 × 01-20; BC 24 ), PO2 (resulting from HE-DGMS87-534 × 87-534; BC 23 ) and PO3 (resulting from HE-DGMS18k × 18k; BC 20 ). Thirty male fertile and thirty male sterile plants were randomly selected from the PO1 population to construct DNA pools. The bulked DNA samples were extracted using a Plant Genomic DNA Kit (Tiangen, Beijing, China), and then sequenced at the Beijing Genomics Institute (BGI) (Beijing, China), with an Illumina Hi-Seq 2500 platform. The resulting data were filtered and aligned to the cabbage reference genome (“02-12” reference genome, version 1). SNP- index and Δ(SNP- index) were calculated. Following the standard protocol for BSA-based mapping, Ms-cd1 was primarily delimited to a genomic interval on C09. A total of 13 markers within the interval were designed using Primer 3 to genotype the plants among the populations. Ms-cd1 was ultimately delimited to a 10.9-kb region. To determine the nucleotide variations between the male-fertile and male-sterile lines, the entire genomic regions were amplified and sequenced from 01-20, HE-DGMS01-20, HO-DGMS01-20, 87-534, HE-DGMS HO-DGMS87-534, 18K and HE-DGMS18K. A list of primers for positional cloning and DNA fragment amplification is shown in Supplementary Data 2 . Plasmid construction and Agrobacterium -mediated plant genetic transformation For functional complementation, a fragment 6028 bp in length containing the mutated promoter region, Ms-cd1 gene coding region and terminator region (340 bp) was amplified from DGMS01-20 genomic DNA and inserted into a modified pCAMBIA1301 vector to generate PΔ-597::gMs-cd1 . To knock out the Ms-cd1 gene, a single guide RNA (sgRNA) sequence (5’-ACGATGCATCGCACAAGAAAGGG-3’) targeting the Ms-cd1 coding region was designed and inserted into a modified pKSE401 CRISPR/Cas9 plasmid to generate Ms-cd1 -CRISPR/Ca9. To knock out the BoERF1L gene, a sgRNA sequence (5’-ATTATGTACAGCTACGAGGATGG-3’) targeting the BoERF1L coding region was designed and inserted into a modified pKSE401 CRISPR/Cas9 plasmid to generate BoERF1L -CRISPR/Ca9. For BoERF1L gene RNAi, a 202-bp specific fragment of the BoERF1L coding sequence (44–245 bp) was synthesized and inserted into a pFGC5941 vector to generate a BoERF1L -RNAi construct. To generate a PΔ-597::Ms-cd1 construct, the mutated Ms-cd1 promoter (amplified from PΔ-597::gMs-cd1 ) and Ms-cd1 CDS were cloned and inserted into a modified pCAMBIA1301 vector. All plasmids contained Bar , Hyg or Kana resistance genes for selection during Agrobacterium -mediated transformation. All plasmids were verified by Sanger sequencing at Tsingke Biological Technology (Beijing, China) and transformed into Agrobacterium strain GV3101. PΔ-597::gMs-cd1 , BoERF1L -RNAi and BoERF1L -CRISPR/Ca9 were transformed into the cabbage inbred line 01-20. Ms-cd1 -CRISPR/Cas9 was used to transform 01-20 and DGMS01-20. PΔ-597::Ms-cd1 was used to transform A. thaliana Col-0, rice ZH11, tomato Ailsa Craig and rapeseed Westar. Agrobacterium -mediated transformation in cabbage, rice, rapeseed, tomato and A. thaliana was performed using a standard protocol [39] , [40] , [41] , [42] . For genetic transformation in cabbage, hypocotyls from 6-day-old seedlings were cut into 0.8–1 cm explants and precultured for 2 days, and then inoculated and cocultured with Agrobacterium tumefaciens strain GV3101 carrying the target vector. After cocultivation for 2 days, the explants were transferred to selection medium (4.43 g/L MS + 0.1 mg/L 1-naphthaleneacetic acid + 1 mg/L 6-bnzylaminopurine + 30 g/L sucrose + 12 mg/L Basta + 300 mg/L Timentin + 0.8% agar; pH: 5.84–5.90). Basta-resistant shoots were obtained under this selection culture. The resulting transgenic plants were identified via PCR amplification in conjunction with primers for Bar , HYG or Kana . At least 5 independent lines were generated for each transformation. To identify the plants with edited genes, the target gene was amplified from genomic DNA and sequenced to search for insertions/deletions within the target site. Quantitative real-time PCR (qRT‒PCR) analysis Total RNA was extracted from various cabbage tissues, including roots, stems, leaves, floral buds and anthers, at different stages using an RNAprep Pure Plant Kit (Tiangen, Beijing, China). First-strand cDNA was synthesized using a PrimeScript 1st Strand cDNA Synthesis Kit (Tiangen, Beijing, China) following the protocols described by the supplier. qRT‒PCRs were performed using SYBR Premix Ex Taq II (Tli RNase H Plus; Takara) on a CFX96 Touch Real-Time PCR Detection System (Bio-Rad, Hercules, CA, USA). The B. oleracea Actin gene ( AF044573.1 ) and Arabidopsis Actin gene ( AT5G09810.1 ) were used as reference controls. Each sample involved assaying three biological replicates, and there were three technical repeats. The data were analyzed by the 2 −ΔΔCT method [43] , and the relative expression levels are given as the means ± SDs. The primers used for qRT‒PCR are listed in Supplementary Data 2 . Promoter‒GUS analysis The WT promoter (PWT) and mutated promoter (PΔ-597) of Ms-cd1 were amplified from 01-20 and HO-DGMS01-20, respectively, inserted into a modified pCAMBIA1301 vector in place of the CaMV 35S promoter and fused to a GUS reporter gene. The generated PWT::GUS and PΔ-597::GUS plasmids were verified via Sanger sequencing and transformed into A. thaliana . The transgenic plants were germinated on 1/2-strength Murashige and Skoog media supplemented with 30 mg/L hygromycin B, and the presence of the HYG gene was verified via PCR. At least 20 independent lines were generated for PWT::GUS and for PΔ-597::GUS . From the T2 generation, ten PWT::GUS lines and ten PΔ-597::GUS lines were randomly selected for histochemical GUS staining. Arabidopsis tissues were fixed in 90% (v/v) acetone and washed with GUS staining buffer (50 mM sodium phosphate buffer, pH 7.2, 0.2% Triton X-100, 2 mM potassium ferrocyanide, and 2 mM potassium ferricyanide). Then the GUS staining buffer was supplemented with 2 mM X-Gluc (Sigma 203783) until a blue color became visible. The samples were then immersed in 75% (v/v) ethanol to remove chlorophyll. GUS activity was measured by quantitation of 4-methylumbelliferone produced by cleavage of the substrate 4-methylumbelliferyl-b-D-glucuronide (Duchefa) on an F97 pro Fluorometer (Shanghai Lengguang Technology Co., Shanghai, China). qRT‒PCR analysis of the GUS gene was performed using Actin as an internal control. RNA in situ hybridization Floral buds of 01-20 and HE-DGMS01-20 cabbage at different developmental stages were collected, fixed in FAA solution (50% ethanol, 5% acetic acid, 3.7% formaldehyde), and stored at 4 °C overnight. The fixed floral buds were dehydrated through an ethanol solution series of 70%, 80%, 90% and 100% followed by clearing in a xylene solution series of 25%, 50%, 75% and 100% and then embedded in paraffin (Paraplast High Melt, Leica). The samples were cut into 8–10 μm sections using a microtome (RM2255, Leica, Wetzlar, Germany) and then mounted on poly-L-lysine-coated glass slides (P0425-72AE; Sigma‒Aldrich). A 200-bp cDNA fragment from Ms-cd1 was subsequently synthesized and inserted into a pGEM-T Easy vector (Promega, Madison, WI, USA). Digoxigenin (DIG)-labeled sense and antisense probes were produced from T7 and SP6 polymerase using a DIG Northern Starter Kit (12039672910, Roche) following the manufacturer’s instructions. RNA ISH with the sense and antisense probes was performed, observed under a BX-51TRF microscope (Olympus, Tokyo, Japan) and imaged with a microcolor charge-coupled device camera (UCMOS05100KPA, ToupTek Photonics, Hangzhou, China). Subcellular localization analysis of Ms-cd1 To reveal the subcellular localization of Ms-cd1 , we generated a 35S::Ms-cd1-GFP transient expression vector. The coding sequence of Ms-cd1 was fused to the N-terminus of GFP and cloned into and inserted into PC1300. The resulting 35S::Ms-cd1-GFP vector was then transformed into Agrobacterium strain GV3101. Agrobacterium suspensions of 35S::Ms-cd1-GFP and p19 suppressor were mixed together equally, and infiltration suspensions consisting of 10 mM 2-(N-morpholino)ethanesulfonic acid (MES), 10 mM MgCl 2 and 100 mM acetosyringone were prepared. Leaves of tobacco plants were subsequently infiltrated with the suspension. After the leaves were incubated for 18 h in the dark and 24 h under light, the GFP signal in tobacco leaves was excited by a 488-nm laser and detected at 510 nm under a confocal microscope (Carl Zeiss AG, Oberkochen, Germany). Phylogenetic analyses The protein sequences of Ms-cd1 and BoERF1L were used as queries to search for homologs with the BLASTP tool of the NCBI database. Homologous protein sequences were downloaded from the NCBI database, and they were named according to published information or their NCBI accession number. The protein sequences were aligned by ClustalW, and a neighbor-joining phylogenetic tree was constructed with MEGA software (version 7) with the Poisson model and 1000 bootstrap replicates. Information concerning the homologous proteins is shown in Supplementary Data 3 . Y1H assays Cabbage floral buds (<3.5 mm) were collected for cDNA library construction via a Matchmaker GAL4 One-Hybrid System (Clontech) following the manufacturer’s instructions. A 66-bp fragment (624–559 upstream of ATG) from the WT promoter was synthesized by staff at BGI Tech (Beijing, China) and subcloned and inserted into a pAbAi vector, and the resulting pABAi-WTpro bait was transformed into the yeast strain Y1HGold. Y1H library screening assays were performed against the cDNA expression library using the Matchmaker GAL4 One-Hybrid System (Clontech). Competent Y1HGold yeast cells containing pABAi-WTpro as bait were transformed with the contents of the cDNA library, plated onto selective SD/-Leu media supplemented with 200 ng/mL AbA, and incubated at 30 °C. The p53-AbAi Control Vector and p53 Control Insert from Clontech were used as the controls. Yeast plasmids from positive colonies were extracted from positive colonies and transformed into Escherichia coli DH5α competent cells. The prey fragments from the positive colonies were identified by Sanger sequencing. To verify the interaction of BoERF1L with the bait, the full-length cDNA sequences of BoERF1L were amplified and fused in frame with the GAL4 activation domain of pGADT7rec (Clontech), forming pGADT7-BoERF1L. In addition to the pABAi-WTpro reporter, we constructed another reporter, pABAi-MTpro, with a 65-bp fragment (624–559 upstream of ATG) from the DGMS01-20 promoter inserted into the pAbAi vector. The pGADT7-BoERF1L construct was subsequently cotransformed with the reporter vectors. DNA‒protein interactions were determined according to the growth of the transformants on SD/-Leu media supplemented with 200 ng/mL AbA. Electrophoretic mobility shift assay For expression and purification of the His-BoERF1 recombinant protein, the full-length coding sequence of BoERF1 was fused to a His tag at the C-terminus and then subcloned and inserted into a pET-SUMO vector. The resulting construct was transformed into E. coli Rosetta (DE3) cells, and the transformed bacteria were cultured in Luria–Bertani media supplemented with 100 mg/mL Kana at 37 °C. Expression of fusion proteins was induced overnight at 30 °C by the addition of 0.1 mM isopropyl b-D-1-thiogalactopyranoside. Recombinant His-BoERF1 was subsequently purified using glutathione-agarose beads (BD Biosciences) according to the manufacturer’s instructions. EMSAs were conducted following the manufacturer’s instructions. Briefly, biotin-labeled and unlabeled Ms-cd1 promoter probes were synthesized by Sangon Biotech (Shanghai, China). The purified BoERF1-His protein and biotin-labeled probes were incubated in a 10 µL reaction mixture that included 2 μg of recombinant protein, 20 fmol of biotin-labeled DNA and 2 µL of 5× EMSA/Gel-Shift Binding Buffer (GS005, Beyotime). The products were analyzed using 6% polyacrylamide gels. To verify binding specificity, 20-, 30- and 40-fold excesses of unlabeled DNA probe were added, and the His-BoERF1 protein was used as a negative control. Dual-LUC transient expression assays The 2.9-kb promoter region of Ms-cd1 PWT was amplified from PWT::GUS via PCR and cloned and inserted into a pluc-35Rluc transient expression vector [44] to generate a PWT::LUC plasmid used as a reporter. The BoERF1L coding sequence was subsequently amplified via PCR from the 35S::Ms-cd1 vector and cloned and inserted into a pCAMBIA 2300 vector to generate the 35S::BoERF1L effector plasmid. An empty pluc-35Rluc construct was used as a negative control. The plasmids were transformed into A. tumefaciens strain EHA105. Agrobacterium cells carrying the effector, reporter and p19 plasmids were suspended using 10 mM MgCl 2 and 150 μM acetosyringone and mixed in a volume ratio of 2:1:3. The suspensions were infiltrated into leaves of 5–6-week-old tobacco plants using a syringe. The leaves were sampled 48 h after infiltration. Firefly luciferase and Renilla luciferase activities were determined using a dual-LUC reporter assay system (E1910, Promega). The results are shown as LUC/REN ratios. Luciferase luminescence was captured using a Tanon 5200 system (Berthold, Tanon, Shanghai, China). Reporting summary Further information on research design is available in the Nature Portfolio Reporting Summary linked to this article.